Coagulase-negative staphylococci release a purine analog that inhibitsStaphylococcus aureusvirulence Coagulase-negative staphylococci and Staphylococcus aureus colonize similar niches in mammals and conceivably compete for space and nutrients. Here, we report that a coagulase-negative staphylococcus, Staphylococcus chromogenes ATCC43764, synthesizes and secretes 6-thioguanine (6-TG), a purine analog that suppresses S. aureus growth by inhibiting de novo purine biosynthesis. We identify a 6-TG biosynthetic gene cluster in S. chromogenes and other coagulase-negative staphylococci including S. epidermidis , S. pseudintermedius and S. capitis . Recombinant S. aureus strains harbouring this operon produce 6-TG and, when used in subcutaneous co-infections in mice with virulent S. aureus USA300, protect the host from necrotic lesion formation. Used prophylactically, 6-TG reduces necrotic skin lesions in mice infected with USA300, and this effect is mediated by abrogation of toxin production. RNAseq analyses reveal that 6-TG downregulates expression of genes coding for purine biosynthesis, the accessory gene regulator (agr) and ribosomal proteins in S. aureus , providing an explanation for its effect on toxin production. Staphylococcus aureus is an opportunistic human pathogen and a significant cause of morbidity and mortality worldwide, causing a wide spectrum of diseases ranging from superficial skin and soft tissue infections to severe life-threatening diseases such as endocarditis and pneumonia [1] , [2] . The enormous health burden caused by S. aureus is, in part, attributed to its ability to acquire resistance against several classes of antibiotics, making it refractory to many treatment options. Moreover, methicillin-resistant S. aureus (MRSA) can infect both healthy and immunocompromised populations in the community and hospital setting [3] , [4] , [5] . Due to the emergence of MRSA, drug discovery is critically important for combating S. aureus infections [6] , [7] . To identify compounds that antagonize S. aureus , several groups have focused on coagulase-negative staphylococcal species (CoNS) as many of these species often colonize the same niches as S. aureus and likely compete for space and nutrients [8] , [9] , [10] . To successfully compete with S. aureus , CoNS have been shown to secrete antimicrobials that directly kill S. aureus [10] , [11] . Indeed, strains of S. epidermidis and S. hominis species, among others, have been reported to secrete posttranslationally modified peptides termed bacteriocins that inhibit S. aureus colonization on human skin [11] . In addition, S. lugdunensis has recently been shown to produce the non-ribosomally synthesized cyclic peptide antibiotic termed lugdunin that directly kills S. aureus [10] . Moreover, lugdunin can stimulate host production of antimicrobial peptides and recruit immune cells to clear S. aureus infections [12] . Another strategy used by some CoNS including S. schleiferi and S. caprae is the secretion of autoinducing peptides that specifically block the activation of the agr quorum sensing system in S. aureus . By doing so, these CoNS reduce S. aureus virulence and interfere with colonization of the host [9] , [13] , [14] . Clearly, CoNS have evolved mechanisms to antagonize S. aureus growth and virulence to gain a competitive advantage. S. chromogenes is a CoNS that can secrete antimicrobials to antagonize S. aureus and other bacteria [8] , [15] , [16] , [17] . Here, we show that S. chromogenes ATCC43764 secretes the purine analog 6-thioguanine (6-TG) to impede S. aureus growth. The underlying genetic basis for 6-TG biosynthesis was elucidated in S. chromogenes as a six-gene operon, termed tgs for thioguanine synthesis; the tgs operon was also identified in the genomes of a number of S. capitis , S. pseudintermedius , and S. epidermidis strains. We show that the operon from tgs -positive CoNS strains encodes 6-TG, which is inhibitory to S. aureus . This was shown to be the case in vivo as well, as co-infections of virulent S. aureus USA300 with tgs -positive S. epidermidis or S. aureus RN4220 (a cloning strain) carrying tgs genes on a plasmid demonstrated a significant reduction in skin lesion necrosis. Moreover, 6-TG reduced S. aureus disease severity in a subcutaneous murine infection model, owing to its effect on downregulating toxin production by S. aureus . The therapeutic effects of 6-TG are due to its ability to reduce gene expression of the agr quorum sensing system, ribosomal proteins, and purine biosynthesis. This study identifies a mechanism by which CoNS interfere with growth and virulence of S. aureus . 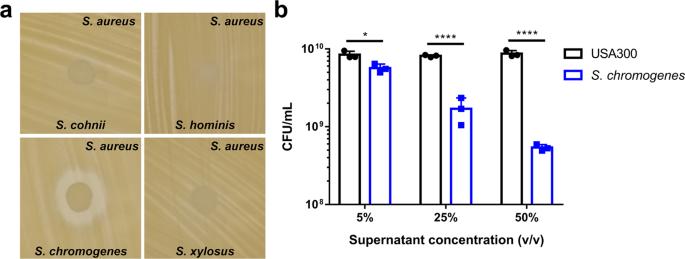Fig. 1:S. chromogenessecretes a molecule that inhibitsS. aureusgrowth. aSimultaneous antagonism assay of selected representative CoNS on TSA.bS. aureuswas cultured in TSB containing spent culture supernatant fromS. chromogenesorS. aureus. The bacteria were grown for 24 h before they were plated and CFU/mL were enumerated. Results are pooled from three independent experiments. Data are shown as mean ± SD (n= 3, *p≤ 0.05, ****p≤ 0.0001. Two-sided unpairedt-test). S. chromogenes ATCC43764 inhibits S. aureus by secreting 6-TG To identify CoNS that antagonize the community-acquired MRSA strain S. aureus USA300-LAC (hereafter termed S. aureus ), we screened a number of CoNS using the simultaneous antagonism assay [3] (Supplementary Table 1 and Fig. 1a ). Among the species and strains screened, we found that S. chromogenes strain ATCC43764, the type strain for the species, inhibited S. aureus growth on tryptic soy agar (TSA). We next demonstrated that the inhibitory molecule was secreted as spent culture supernatant (hereafter termed supernatant) of S. chromogenes also inhibited growth of S. aureus in liquid culture (Fig. 1b ). The secreted molecule with inhibitory activity was found to be <3 kDa and resistant to heat and proteases (Supplementary Fig. 1 A–D). For identification, the active molecule in S. chromogenes supernatant was enriched using sequential steps of centricon filtration, FPLC, and, finally, HPLC. Following HPLC, several contiguous fractions antagonized S. aureus growth equally (Supplementary Fig. 2A ). 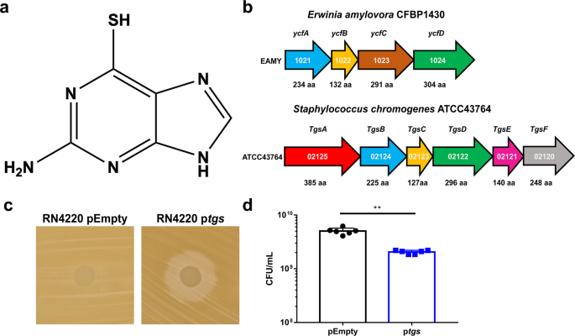Fig. 2: Identification of a 6-TG biosynthetic gene cluster inS. chromogenes. aMolecular structure of 6-thioguanine.bE. amylovora ycfoperon andS. chromogenes6-TG biosynthetic operon.cSimultaneous antagonism assay using RN4220 pEmpty and ptgson TSA.dS. aureuswas cultured in TSB containing supernatant from RN4220 pEmpty or ptgsand plated 24 h.p.i and CFU/mL were enumerated. Results are pooled from two independent experiments, each withn= 3 replicates per condition. Data are shown as mean ± SD (**p≤ 0.01. Two-sided unpairedt-test). These fractions were then analyzed by mass spectrometry in three independent experiments (Supplementary Table 2 ) to identify molecules present. We calculated a “score ratio” of these molecules to determine the relative abundance of these compounds across contiguous fractions within each experiment and found three molecules present in relatively equal abundance in biologically active fractions between experiments. Using these criteria, 6-TG (tioguanine; thioguanine), cinnamic acid, and indoleacrylic acid were the best candidate molecules (Supplementary Table 2 ). Indoleacrylic acid exerts anti-inflammatory activity and promotes intestinal barrier function [18] and, based on this, we surmised it was unlikely to antagonize S. aureus growth. Interestingly, 6-TG and cinnamic acid have previously been shown to inhibit bacterial growth [19] , [20] , [21] . While cinnamic acid had no inhibitory effect on S. aureus , 6-TG impaired S. aureus growth on TSA (Supplementary Fig. 2B ). Taken together these data suggest that the inhibitory molecule secreted by S. chromogenes is 6-TG (Fig. 2a ). Fig. 1: S. chromogenes secretes a molecule that inhibits S. aureus growth. a Simultaneous antagonism assay of selected representative CoNS on TSA. b S. aureus was cultured in TSB containing spent culture supernatant from S. chromogenes or S. aureus . The bacteria were grown for 24 h before they were plated and CFU/mL were enumerated. Results are pooled from three independent experiments. Data are shown as mean ± SD ( n = 3, * p ≤ 0.05, **** p ≤ 0.0001. Two-sided unpaired t -test). Full size image Fig. 2: Identification of a 6-TG biosynthetic gene cluster in S. chromogenes . a Molecular structure of 6-thioguanine. b E. amylovora ycf operon and S. chromogenes 6-TG biosynthetic operon. c Simultaneous antagonism assay using RN4220 pEmpty and p tgs on TSA. d S. aureus was cultured in TSB containing supernatant from RN4220 pEmpty or p tgs and plated 24 h.p.i and CFU/mL were enumerated. Results are pooled from two independent experiments, each with n = 3 replicates per condition. Data are shown as mean ± SD (** p ≤ 0.01. Two-sided unpaired t -test). Full size image Identification of the 6-TG biosynthetic gene cluster in S. chromogenes ATCC43764 Next we sought to determine the genetic basis of 6-TG biosynthesis in S. chromogenes ATCC43764. To date, only Erwinia amylovora , a Gram-negative plant pathogen, has been shown to synthesize 6-TG, attributable to the four-gene ycf operon [22] , [23] . Hence, we sequenced and annotated the S. chromogenes ATCC43764 genome to mine for encoded proteins with predicted functional domains similar to YcfA and YcfB from E. amylovora , which are necessary and sufficient for 6-TG biosynthesis [23] . Using InterPro to predict functional protein domains, we identified Rossman-like alpha/beta/alpha folds and an adenine nucleotide hydrolase-like domain in YcfA and NADH pyrophosphatase and NUDIX hydrolase domains in YcfB. Interestingly, we found two gene products with identical functional domains within a predicted six-gene operon in the S. chromogenes ATCC43764 genome (Fig. 2 b). Examination of the predicted products of each of the six genes within the operon (see Table 1 ) suggest roles in sulfur transfer, nucleotide metabolism, and secretion/efflux. Table 1 Putative function of gene products in the S. chromogenes 6-TG biosynthetic cluster. Full size table To prove this operon in S. chromogenes was responsible for synthesizing 6-TG, we attempted to delete it from the S. chromogenes genome. Unfortunately, we were unable to transform the bacterium using existing plasmids and thus we were unable to genetically modify S. chromogenes using traditional molecular genetic methodologies. In lieu of this, we thus amplified and then cloned the genes from S. chromogenes into a plasmid and introduced this recombinant plasmid into S. aureus RN4220, creating a strain termed RN4220 p tgs . Remarkably, we showed that RN4220 p tgs inhibited S. aureus growth on TSA while RN4220 carrying an empty vector (termed RN4220 pEmpty) did not impair S. aureus growth (Fig. 2c ). Moreover, supernatant from RN4220 p tgs inhibited S. aureus growth whereas supernatant from RN4220 pEmpty did not (Fig. 2d ). Mass spectrometry was used to confirm that supernatants from RN4220 p tgs , but not RN4220 pEmpty, contained 6-TG (Supplementary Fig. 2C ). Taken together, these data identify the genetic basis of 6-TG biosynthesis in S. chromogenes ATCC43764 and confirm that the expression of these genes by this species is detrimental to the growth of S. aureus . The six-gene operon was thus designated tgs A-F , for thioguanine synthesis. Identification of the tgs operon in other staphylococcal species Next, we assessed the diversity of the tgs operon and its homologs in publicly available genomes of Staphylococcus species. We surveyed 1388 genomes across seven different species of Staphylococcus and discovered that the operon and its homologs can be found in genomes from S. capitis , S. chromogenes , S. epidermidis , and S. pseudintermedius (Table 2 and Supplementary Data 1 ). A phylogenetic analysis of these sequences showed that the tgs operon grouped into species-specific clades, suggesting that the operon was acquired by a common ancestor of each species and was then passed down via vertical inheritance (Fig. 3a ). Interestingly, in S. chromogenes strain 1401, the operon is present on a plasmid, suggesting that it has the potential to be passed between different strains and species via horizontal gene transfer. Table 2 The tgs operon among staphylococcal species. Full size table Fig. 3: The tgs operon is present in other staphylococcal species and functional. a Phylogenetic analysis of the 6-TG operon using completed and draft Staphylococcus genomes. Black triangles represent a clade that was collapsed because their internal bootstrap values were <50%. SCa S. capitis , SCh S. chromogenes , SE S. epidermidis , SP S. pseudintermedius . b Simultaneous antagonism assay of tgs -negative and -positive staphylococcal strains on TSA. c Simultaneous antagonism assay using RN4220 pEmpty and pVCU116 tgs on TSA. d S. aureus was cultured in TSB containing supernatant from RN4220 pEmpty or pVCU116 tgs and plated 24 h.p.i and CFU/mL were enumerated. Results are pooled from two independent experiments, each with n = 3 replicates per condition. Data are shown as mean ± SD (** p ≤ 0.01. Two-sided unpaired t -test). Full size image To determine whether other CoNS that encode the tgs operon inhibit S. aureus growth in vitro, we tested both tgs- negative and -positive strains that were identified in our bioinformatic analyses using the simultaneous antagonism assay. As expected, the tgs -positive S. epidermidis M23864:W2 strain inhibited growth of S. aureus while the tgs- negative strains did not. However, both tgs -positive S. capitis strains did not inhibit S. aureus growth in our assay conditions (Fig. 3b ). This result led us to hypothesize that expression of the tgs operon in these strains was repressed. Thus, to test this hypothesis, we amplified and cloned the tgs operon from one of the S. capitis strains (VCU116) into a plasmid, and introduced this recombinant plasmid into S. aureus RN4220, creating a strain termed RN4220 pVCU116 tgs . Of note, RN4220 pVCU116 tgs inhibited S. aureus growth while RN4220 pEmpty did not (Fig. 3 c, d). Mass spectrometry confirmed that both RN4220 pVCU116 tgs and S. epidermidis M23864:W2 produce 6-TG. Moreover, supernatants from both tgs -positive S. capitis strains had detectable levels of 6-TG, although ~20-fold less than that of RN4220 pVCU116 tgs or the other tgs -positive species that showed growth-inhibitory effects on S. aureus (Supplementary Fig. 3A ). Therefore, it is likely that the S. capitis strains did not inhibit S. aureus growth due to low amounts of secreted 6-TG. Next, we assessed whether expression of the tgs operon from both S. chromogenes and S. capitis is detrimental to RN4220, a S. aureus cloning strain. Both RN4220 p tgs and RN4220 pVCU116 tgs show a growth defect compared to RN4220 pEmpty, revealing that 6-TG production is detrimental to the growth of the producing S. aureus strain RN4220 (Supplementary Fig. 3B ). Expression of tgs genes ameliorates S. aureus virulence in vivo Our results demonstrated that staphylococci that express the tgs operon inhibit S. aureus growth in vitro. To determine whether these strains can offer protection to the host and antagonize S. aureus in vivo, we performed co-infection experiments using S. aureus USA300 and tgs -negative or - positive S. epidermidis strains in a subcutaneous infection model, as these species are known to co-colonize on human skin [11] , [24] . We mixed S. aureus with either a tgs -negative or - positive S. epidermidis strain in a 1:1 ratio and measured the size of lesions over time. Importantly, we observed that co-infections with a tgs- positive S. epidermidis strain reduced skin damage caused by S. aureus compared to co-infections with a tgs -negative S. epidermidis strain (Fig. 4a, b ). Admittedly, these experiments using different S. epidermidis strains were correlative. However, to demonstrate a causative effect of tgs genes, we repeated these co-infection experiments by combining S. aureus USA300 (produces necrotic lesions) with S. aureus RN4220 (does not produce necrotic lesions) carrying either pEmpty or p tgs . Remarkably, we observed that co-infections with RN4220 p tgs resulted in significantly smaller lesions compared to co-infections with RN4220 pEmpty (Fig. 4c, d ). These data show that staphylococci that express the tgs operon can protect the host against necrotic skin infections caused by S. aureus . Fig. 4: tgs expressing staphylococci reduce skin damage caused by S. aureus during co-infection. a Representative images showing necrotic skin lesions 4 days post infection with S. aureus + tgs- negative S. epidermidis str. VCU036 or S. aureus + tgs -positive S. epidermidis str. M23864:W2 in a 1:1 ratio. b Quantitation of necrotic skin lesion size 4 days post infection with S. aureus + tgs -negative S. epidermidis str. VCU036 or S. aureus + tgs -positive S. epidermidis str. M23864:W2 in a 1:1 ratio. Results are from one representative experiment enumerating 8 lesions per group ( n = 4 animals per group). Data are shown as mean ± SD (*** p ≤ 0.001. Two-sided unpaired t -test). c Representative images showing necrotic skin lesions 4 days post infection with S. aureus + RN4220 pEmpty or S. aureus + RN4220 p tgs in a 1:1 ratio. d Quantitation of necrotic skin lesion size 4 days post infection with S. aureus + RN4220 pEmpty or S. aureus + RN4220 p tgs in a 1:1 ratio. Results are from one experiment enumerating 8 lesions per group ( n = 4 animals per group). Data are shown as mean ± SD (*** p ≤ 0.001. Two-sided unpaired t -test). Full size image 6-TG inhibits tissue necrosis during subcutaneous S. aureus infection Although co-infections with tgs -positive strains can protect the host against skin damage caused by S. aureus , it is unlikely that these strains can be administered as a probiotic to combat S. aureus infections as these bacteria may also cause infections on their own. Therefore, we sought to assess the therapeutic effect of 6-TG on formation of necrotic skin lesions in a subcutaneous S. aureus infection. To do this, we prophylactically administered 6-TG subcutaneously and measured the size of lesions throughout infection. Strikingly, we observed that the necrotic lesions of treated mice were significantly smaller than the lesions on mice injected with vehicle control (Fig. 5a, b ). Moreover, we observed a reduction in bacterial load when we excised the lesions of mice treated with 6-TG relative to the mice given the vehicle control (Supplementary Fig. 4 ). However, in additional and in subsequent experiments, and irrespective of lesion size, if we excised similar areas of skin from both the vehicle and 6-TG-treated mice we found that, despite significant differences in lesion size between treated vs. untreated groups, similar bacterial burdens were present at 4 days post infection (Fig. 5c ). The discrepancy in the measured bacterial load using these two methods suggest that quantification of CFUs is more accurate when a large section of the skin is excised, irrespective of the lesion size. Taken together, these data demonstrate that prophylactic treatment with 6-TG significantly reduces necrotic lesion formation caused by S. aureus . Fig. 5: Prophylactic treatment with 6-TG reduces necrotic lesion size in subcutaneous infection. a Representative images showing necrotic skin lesions 4 days post infection with S. aureus ± prophylactic 6-TG treatment. b Quantitation of necrotic skin lesion size 4 days post infection with S. aureus ± prophylactic 6-TG (20 µg) treatment. Results are pooled from two independent experiments with 8–12 lesions per group ( n = 4 and 6 animals, respectively). Data are shown as mean ± SD (**** p ≤ 0.0001. Two-sided unpaired t -test). c Skin tissue was excised from mice infected with S. aureus 4 days post infection ± prophylactic 6-TG treatment (20 µg) and plated onto TSA to enumerate CFUs. Results are from one experiment with 8–12 lesions per group ( n = 4 and 6 animals, respectively). Data are shown as mean ± SD (two-sided unpaired t -test). Full size image 6-TG blocks toxin production in S. aureus in a purine-dependent and -independent manner 6-TG is a guanine analog that is known to inhibit purine biosynthesis [20] , [25] . In support of the notion that 6-TG inhibits S. aureus growth by interfering with purine biosynthesis, we show that a S. aureus purK mutant, with a disrupted purine biosynthesis pathway [26] , was largely resistant to 6-TG-mediated growth inhibition on TSA (Supplementary Fig. 5A ). Furthermore, 6-TG is more potent against S. aureus grown on purine-deplete RPMI than on TSA (Supplementary Fig. 5A, B ). Indeed, S. aureus growth was partially rescued by addition of guanine in RPMI (Supplementary Fig. 5B ). Interestingly, 6-TG is also active against strains representing other S. aureus clonal lineages, although to varying degrees (Supplementary Fig. 6 ). Taken together, these data indicate that 6-TG primarily impairs S. aureus growth by inhibiting purine biosynthesis. Since 6-TG abrogated necrosis in the S. aureus subcutaneous infection model, we questioned whether the compound could curtail production of S. aureus secreted toxins, which are required for tissue necrosis in this model [27] . Interestingly, several studies demonstrate a link between purine biosynthesis and S. aureus virulence [20] , [26] , [28] , [29] , [30] , [31] . To determine whether 6-TG, a purine biosynthesis inhibitor, reduces toxin production, we cultured S. aureus in tryptic soy broth (TSB) with 6-TG or a vehicle control to stationary phase (OD 600 = 7.0), collected supernatants and analyzed the secreted protein profile using SDS-PAGE. We observed that supernatants from bacteria grown with 6-TG had less overall protein, including several toxins, compared to vehicle treated cultures (Fig. 6a ). Next, we chose Hla as a representative S. aureus toxin and evaluated the effects of 6-TG on its levels in S. aureus cultures. Importantly, this toxin is known to be important for S. aureus pathogenesis in skin infections [27] , [32] , [33] . Here, we used an anti-Hla antibody to confirm that Hla levels were dramatically reduced when S. aureus was exposed to 6-TG (Fig. 6b ), and demonstrated that this reduction in Hla was dose-dependent and correlated with its effect on growth (Supplementary Fig. 7A–C ). Fig. 6: 6-TG reduces S. aureus toxin production in a purine-dependent and -independent manner. a S. aureus was grown in the presence of 6-TG (10 µg/mL) or a vehicle control to an OD 600 of 7.0 and secreted proteins in the supernatant were TCA precipitated and separated by SDS-PAGE. This experiment was repeated three times with similar results. b Protein samples in a were immunoblotted and probed with anti-alpha toxin antibody in a Western blot. Protein identification was by MALDI TOF MS. Numbers indicate molecular mass markers. This experiment was repeated three times with similar results. c S. aureus and S. aureus purK ::ΦΝΣ was grown in TSB with 6-TG (10 µg/mL) or a vehicle control to an OD 600 of 7.0 and secreted proteins in the supernatant were TCA precipitated and separated by SDS-PAGE. This experiment was repeated twice with similar results. d Protein samples in c were immunoblotted and probed with anti-alpha toxin antibody in a Western blot. This experiment was repeated twice with similar results. e Quantitation of necrotic skin lesion size 4 days post infection with S. aureus or S. aureus purK ::ΦΝΣ ± prophylactic 6-TG (20 µg) treatment. Results are from one representative experiment with 16 lesions enumerated per group ( n = 8 animals). Data are shown as mean ± SD (*** p ≤ 0.001, ** p ≤ 0.01, * p ≤ 0.05. Two-sided unpaired t -test). f Skin tissue was excised from mice infected with S. aureus or S. aureus purK ::ΦΝΣ 4 days post infection ± prophylactic 6-TG (20 µg) treatment and plated onto TSA to enumerate CFUs. Results are from one representative experiment with 16 lesions enumerated per group ( n = 8 animals). Data are shown as mean ± SD (*** p ≤ 0.001. Two-sided unpaired t -test). For a–d , numbers to the left of gels/blots are molecular mass markers (in kDa). Full size image To determine whether toxin production was abrogated by 6-TG due to its effect on purine biosynthesis, we performed SDS-PAGE on culture supernatants from S. aureus and purK ::ΦΝΣ grown in TSB with 6-TG or a vehicle control. Interestingly, we observed that purK ::ΦΝΣ secretes less overall protein compared to its wild-type counterpart in the absence of 6-TG, confirming that purine biosynthesis is linked to toxin production in S. aureus . However, purK ::ΦΝΣ secretes less overall protein when cultured with 6-TG despite already being deficient in purine biosynthesis (Fig. 6c ). A western blot analysis demonstrated that these findings also extend to Hla protein levels in cell culture supernatants (Fig. 6d ). We confirmed that the effects of 6-TG on purK ::ΦΝΣ were not due to an effect on growth, as the compound does not affect the mutant’s growth kinetics (Supplementary Fig. 8 ). Overall, these results suggest that 6-TG affects toxin production in both a purine-dependent and -independent manner. Next, we evaluated the importance of S. aureus purine biosynthesis for necrotic lesion formation in a subcutaneous infection. Here, we prophylactically treated mice with 6-TG or a vehicle control before subcutaneously infecting them with S. aureus or purK ::ΦΝΣ. As expected, purK ::ΦΝΣ caused smaller necrotic lesions compared to wild-type S. aureus in mice given a vehicle control (Fig. 6e ). However, the lesion size caused by this mutant was unaffected by 6-TG, suggesting that a very-low amount of Hla is required for lesion formation and a significant increase in Hla levels is required to increase lesion size (i.e., the relationship between Hla levels and lesion size is not completely linear). Interestingly, purK ::ΦΝΣ treated with 6-TG had a slight increase in bacterial burden relative to the control without treatment (Fig. 6 f). These data reveal the importance of purine biosynthesis for the regulation of toxin production in S. aureus in a subcutaneous infection model. 6-TG abolishes transcription of ribosomal genes and genes of the pur and agr operons Next, we wanted to determine the exact changes that 6-TG exerts on S. aureus and to understand how it affects toxin production in both a purine-dependent and -independent manner. To accomplish this, we cultured both wild-type S. aureus and its purK ::ΦΝΣ derivative to exponential phase (OD 600 = 1.0) and exposed them to 6-TG for 1 h before collecting the cells and extracting the RNA to perform RNA sequencing (RNA-seq). Some of the most upregulated genes upon exposure to 6-TG were CodY-regulated genes, such as branched chain amino acid synthesis genes. We attribute this to the effects 6-TG has on repressing guanine levels and, thus, guanosine triphosphate (GTP), which is an effector molecule of CodY DNA binding and thus its transcriptional repression [34] . However, to understand how 6-TG inhibits toxin production in S. aureus , we focused our analyses on transcripts that were repressed by 6-TG. As expected, transcripts from the pur operon were significantly downregulated in wild-type cells treated with 6-TG, owing to the drug’s effect on purine biosynthesis. Surprisingly, transcripts from the agr operon and over 40 genes that encode for ribosomal proteins were also significantly reduced by 6-TG in wild-type cells (Fig. 7a ). These results suggest that 6-TG abrogates toxin production in S. aureus in two ways; it downregulates transcription from the global virulence regulator agr and it globally reduces protein synthesis by preventing ribosomal proteins from being synthesized, which consequently impedes toxin production. Indeed, 1-h treatment with 6-TG already reduces the expression of hla by 1.65-fold (40%) (Supplementary Data 2 ). To determine which effects are purine-dependent or -independent, we compared transcript levels between WT and purK ::ΦΝΣ in cultures treated and untreated with 6-TG (Fig. 7b ). Strikingly, there was a strong overlap in genes that were affected by the purK mutation in S. aureus (Fig. 7b ), versus WT treated with 6-TG (Fig. 7a ). Indeed, there was a significant reduction in transcripts from the pur operon because purK ::ΦΝΣ is inherently deficient in purine synthesis. However, the number of transcripts from genes that encode for many ribosomal proteins was also reduced compared to wild-type cells, suggesting a link between purine biosynthesis and ribosome synthesis. Interestingly, transcripts from the agr operon are reduced to a lesser extent in the purine biosynthesis mutant compared with WT that has been treated with 6-TG (Fig. 7b, c.f. a ), suggesting that the effects 6-TG has on agr are not fully purine-dependent. In support of this, transcripts from agr are reduced further when the purK ::ΦΝΣ culture is treated with 6-TG relative to the untreated purK ::ΦΝΣ culture (Fig. 7c ). No significant differences in the number of transcripts were found when comparing the transcriptome of the purK ::ΦΝΣ mutant and wild-type cells when both cultures were treated with 6-TG (Fig. 7d ). Altogether, these data show that 6-TG drastically reduces ribosome synthesis in a purine-dependent manner and blocks agr activation in both a purine-dependent and -independent manner. As a result, production of proteinaceous toxins will be significantly diminished as translation is blocked by 6-TG. Fig. 7: 6-TG abrogates toxin production by reducing transcription from the agr locus and from genes encoding for ribosomal proteins. a RNA-seq analysis of wild-type S. aureus cultures treated with a vehicle control or 6-TG (10 µg/mL) in TSB. Data points above the dashed lines along the x -axis represent p ≤ 0.01. Data points outside of the dashed lines along the y -axis represent fold changes of ≥2.0. Results are from four independent experiments. b RNA-seq analysis of S. aureus purK ::ΦΝΣ cultures treated with a vehicle control compared to wild-type S. aureus cultures treated with a vehicle control in TSB. Results are from four independent experiments. c RNA-seq analysis of S. aureus purK ::ΦΝΣ cultures treated with a vehicle control or 6-TG (10 µg/mL) in TSB. Results are from four independent experiments. d RNA-seq analysis of wild-type S. aureus cultures and S. aureus purK ::ΦΝΣ cultures treated with 6-TG (10 µg/mL) in TSB. Results are from four independent experiments. Statistical significance was determined using a negative binomial distribution. Detailed RNA-seq data can be found in Supplementary Data 2 . Full size image S. aureus is a major human pathogen that causes a spectrum of mild to severe diseases, including self-limiting skin infections to sepsis [1] . The emergence of MRSA has sparked interest in discovering new drugs to combat drug-resistant S. aureus infections. Attention has been focused on CoNS for drug discovery as these species compete against S. aureus in their respective ecological niches. Indeed, CoNS including S. epidermidis, S. hominis, S. lugdunensis , and S. capitis , have been reported to secrete effector molecules to inhibit S. aureus colonization and reduce its virulence [9] , [10] , [11] , [35] . These studies illustrate the importance of CoNS as a potential source of compounds that can be used to treat S. aureus infections. In this work, we found a strain of S. chromogenes that blocks purine biosynthesis to inhibit S. aureus growth. Importantly, de novo purine biosynthesis has recently been shown to regulate the virulence potential of S. aureus [26] , [30] , [31] . It is interesting that the tgs operon was found in S. chromogenes because this is a species that co-colonizes with S. aureus in cattle [36] , [37] , [38] . Since these two species occupy the same ecological niche, it is conceivable that they are in constant competition for space and nutrients. Indeed, it has been suggested that the presence of S. chromogenes offers protection against S. aureus infections in bovines [36] . The conservation of the tgs operon in S. chromogenes and other CoNS suggests that the genes have moved during competition in niches they co-occupy. For example, the CoNS that harbor the tgs operon colonize skin and mucosal surfaces of various mammals including humans, similar to S. aureus and are known to cause opportunistic infections [24] , [39] , [40] . The tgs -positive S. chromogenes and S. epidermidis strains that inhibit S. aureus growth produce at least tenfold more 6-TG into the culture supernatant than the two tgs -positive S. capitis strains. This difference would appear to account for the observed difference in the growth-inhibitory ability between the species, since the S. capitis tgs genes produce enough 6-TG to inhibit S. aureus growth when they are expressed from a multi-copy plasmid. Our ongoing studies seek to define the regulatory mechanism and signal(s) controlling expression of the operon in S. capitis . Here, we showed that NUDIX domain-containing proteins are responsible for 6-TG biosynthesis. NUDIX domain proteins are widespread among microbes and have been implicated in bacterial pathogenesis [41] . Therefore, it is likely that microbes besides Erwinia and staphylococcal species also synthesize 6-TG. At this time, the enzymatic reactions required to synthesize 6-TG are unknown without confirmation of biochemical activity of the Tgs enzymes. Our bioinformatic analyses (Table 1 ) allow us to speculate that GTP can serve as an initial substrate. A combination of TgsC, TgsE, and/or TgsF may cleave the phosphates off GTP to generate guanosine. TgsA is predicted to release a sulfur group from a donor molecule (e.g., cysteine), which then likely serves as a substrate for TgsB, which we predict transfers it guanine. TgsD is a predicted efflux membrane protein and presumably exports 6-TG out of the cell, and likely also therefore provides self-resistance to the molecule. Interestingly, our data demonstrate that, despite possessing the tgsD gene, growth of recombinant S. aureus carrying the tgs operon is still slowed in comparison to strains carrying vector alone (Supplementary Fig. 3 ). In this work, we show that bacteria expressing the tgs operon can reduce lesion formation in a subcutaneous S. aureus infection in a 6-TG-dependent manner during a co-infection. These data along with other studies demonstrate that CoNS on the skin can provide protection against infections caused by the more pathogenic S. aureus on the skin [9] , [11] , [14] . To demonstrate the therapeutic potential of 6-TG, we showed that the pure compound can be used to prophylactically treat S. aureus skin infections. Our data suggest that 6-TG acts therapeutically by reducing the overall amount of toxin that S. aureus may secrete during infection. We show that the molecular basis for the therapeutic effect of 6-TG is likely due to its ability to abrogate purine biosynthesis, which subsequently reduces ribosome synthesis and toxin production. Moreover, 6-TG downregulates transcription of the global virulence regulator agr , further reducing toxin production. By inhibiting de novo purine biosynthesis, we show that 6-TG can act as an anti-virulence compound in a subcutaneous S. aureus skin infection model as purine synthesis and toxin production are linked. These data reveal purine biosynthesis as an attractive drug target for treatment of MRSA infections, as targeting this pathway significantly affects toxin production, which is important for many types of S. aureus infections at different sites of the body [42] . Thus, it will be interesting to determine whether 6-TG can also be used to reduce disease severity and/or bacterial burden in other models of infection in future studies. Indeed, Lan et al. have shown that 6-TG can reduce S. aureus burden in a systemic infection in mice [20] . Moreover, it will be important to test other nucleobase analogs against S. aureus to potentially expand our repertoire of antimicrobials and/or anti-virulence compounds to treat MRSA infections. Like other thiopurines, 6-TG is a pro-drug that enters the purine salvage pathway and is converted into its active form, 6-thioguanosine monophosphate, by the enzyme hypoxanthine-guanine phosphoribosyl transferase (HPRT) in humans [43] . Once converted into an active metabolite, 6-TG is thought to block purine synthesis and be incorporated into DNA, causing cytotoxic effects in eukaryotic cells [25] , [44] . Whether 6-TG affects bacteria by exerting mutagenic effects is currently unknown. However, Sun et al. showed that 6-TG interacts with Mycoplasma pneumoniae HPRT to block purine salvage [21] . This suggests that 6-TG may also antagonize S. aureus through the purine salvage pathway by being activated by HPRT. We are currently investigating the molecular targets of 6-TG and to identify determinants that make S. aureus susceptible to 6-TG. It is well known that certain antibiotics can select for agr mutations and S. aureus strains harboring these mutations become more resistant to these stresses and cause chronic infections [45] . However, we currently have no evidence to suggest that 6-TG selects for the emergence of these mutants or that agr -negative strains are resistant to 6-TG. In this study, we observed that the agr -negative strain RN4220 is susceptible to the growth-inhibitory effects of 6-TG. Future work will seek to identify mechanisms of resistance against 6-TG in S. aureus and how evolving resistance against this drug affects S. aureus physiology and metabolism. It is becoming increasingly clear that many CoNS, including the species identified in this study that contain the tgs operon, co-colonize with S. aureus and competition between these species for the same niches can provide protection for the host. This work reveals a previously unknown mechanism by which the relatively understudied CoNS can inhibit growth and virulence of more pathogenic bacteria like S. aureus . This, in turn, should spark interest in the discovery of additional genes synthesizing other nucleotide analogs that may be used by bacteria in inter-species bacterial warfare. Bacterial strains and plasmids Bacterial strains and plasmids are listed in Supplementary Table 1 . Unless otherwise noted, strains were cultured at 37 °C with 200 RPM shaking. E. coli was grown in Luria broth (LB) or on LB agar containing 100-μg/mL ampicillin to maintain plasmids when necessary. S. aureus USA300 and RN4220 were grown in TSB or on TSB agar plates (TSA). Staphylococcal plasmids were maintained with growth in 10-μg/mL chloramphenicol when necessary. Bacterial supernatant growth inhibition assays Overnight cultures of S. chromogenes and S. aureus were grown in TSB for ~24 h. Cultures were pelleted at 21,000 g for 5 min and supernatants were filter-sterilized using a 0.22μm syringe filter. The OD 600 of S. aureus cultures was normalized to 1.0 and 10 μl (corresponding to 0.01 ODU, ~5 × 10 6 CFUs) were grown in a 1.0-mL mixture of TSB and either S. chromogenes or S . aureus spent culture supernatants (as indicated in figure or legend) in 13-mL tubes at 37 °C with 200 RPM shaking for 24 h. Bacterial cultures were serially diluted and plated onto TSA to enumerate CFUs at 24 h post inoculation. S. chromogenes supernatant treatments For the use of Amicon ® Ultra centrifugal filter units, filter-sterilized supernatants were centrifuged at 3620 g for 20 min to separate the supernatant into filtrate and concentrate. TSB was added to increase the concentrate volume to the original volume of the supernatant. For heat treatment, supernatants were filter-sterilized and incubated in a 95 °C heat block for 1 h. For proteinase K treatment, 10 μL of a 20-mg/mL proteinase K solution was added to 1 mL of filter-sterilized supernatant and incubated in a 37 °C heat block for 1 h. Proteinase K was inactivated at 95 °C for 30 min. For trypsin treatment, 20 μL of a 20-mg/mL trypsin solution was added to 1 mL of filter-sterilized supernatant and incubated in a 37 °C heat block for 1 h. Trypsin was inactivated at 95 °C for 30 min. Fast protein liquid chromatography Twenty milliliter of S. chromogenes <3-kDa supernatant was loaded on a Sigma-Aldrich HiTrap ® SP Fast Flow column on an Amersham Pharmacia Biotech AKTA FPLC system. Samples were eluted in a 0–50% gradient of solvent B (50-mM Tris pH 8.0) over solvent A (20-mM Tris pH 7.5). Five milliliter fractions were collected at a flow rate of 2.0 mL/min. High performance liquid chromatography Ten milliliter of the active fraction from FPLC was concentrated using a SpeedVac vacuum concentrator and re-suspended in 300-μl ddH 2 O. Two hundred microliter of the suspension was injected into a preparative Waters Bondapak C18 column on a Waters Breeze HPLC. Samples were eluted in a 0–100% gradient of solvent B (methanol or acetonitrile) over solvent A (water or water with 0.1% trifluoroacetic acid). Two milliliter fractions were collected at a flow rate of 4.0 mL/min. Liquid chromatography–mass spectrometry for identification of compounds A 10-μl injection of each fraction was eluted from a Thermo Scientific Hypersil Gold C18 column at 40 °C on a Thermo Scientific Ultimate 3000 UHPLC, with a binary solvent system containing water with 0.1% (v/v) formic acid (solvent A) and acetonitrile containing 0.1% (v/v) formic acid (solvent B) at a 0.3-mL/min flow rate. The gradient initiated with a 1.0-min hold at 5% B. From 1.0 to 7.0 min, the gradient increased linearly to 98% B followed by a hold for 3 min. The gradient then decreased linearly to 5% B from 10–10.5 min and held at 5% B for 4.5 min. The Thermo Scientific Q Exactive mass spectrometer was operated using the following settings: Ion source, HESI II; spray voltage, 3.5 kV; sheath gas flow, 15; auxiliary gas, 5; spare gas, 2; capillary temperature, 320 °C; S-lens RF level, 50. A scan range of 100–1200 was used to identify ions in both positive and negative modes. An untargeted MS 2 experiment was performed using an isolation window of 1.0 m / z and a normalized collision energy of 30 (arbitrary units). Untargeted data processing was done using Thermo Compound Discoverer 2.1. Identification of candidate inhibitory compounds Each compound identified using mass spectrometry in every fraction was given a score based on its abundance in their respective fractions; a higher score signifies higher abundance. Compounds were not considered if they were not identified in all three experiments. Next, we divided the score from the fraction with the highest score (i.e., most concentrated) by the one with the lowest score (i.e., least concentrated) for each compound. The formula for each compound was calculated as follows: score ratio = (compound A highest score)/(compound A lowest score). A score ratio of a molecule approaching a value of 1 signifies an equal distribution of that compound between active fractions. Here, we chose to consider hits with a score ratio of 10 or less in all three experiments as potential candidates for the inhibitory molecule. We chose this cut-off for the score ratio under the assumption that the inhibitory compound was evenly distributed throughout the active fractions since inhibitory activity was equal between these fractions. Whole-genome sequencing of genomic DNA S. chromogenes genomic DNA was isolated by phenol–chloroform extraction. The extracted genomic DNA for H278Tor was tagmented using the Nextera XT tagmentation kit (Illumina) according to manufacturer protocol. The tagmented products were sequenced on an Illumina MiniSeq with paired-end sequencing (2 × 150 bp) at the University of Toronto. The extracted genomic DNA for H278Pit, H279, JB98, and JB383 was tagmented using the Nextera tagmentation kit (Illumina) using a modified protocol [46] . The tagmented products were sequenced on an Illumina NextSeq 550 with paired-end sequencing (2 × 150 bp) at the Microbial Genome Sequencing Center in Pittsburgh, PA. The “Pit” and “Tor” designations for H278 refer to the sequencing location for the isolates to differentiate between the two during downstream analyses. DNA sequence reads were trimmed using Trimmomatic version 0.36 [47] with the following parameters: ILLUMINACLIP, NexteraPE:2:30:10:8:true; LEADING, 20; TRAILING, 20; SLIDINGWINDOW, 4:20; MINLEN, 36. The reads were assembled using the SPAdes version 3.13 assembler [48] in careful mode. Contigs for both the whole genome and the plasmid were annotated using Prokka version 1.12 [49] . Bioinformatic analyses of the 6-TG operon in Staphylococcus species Draft and completed genomes of seven different Staphylococcus species ( capitis , caprae , chromogenes , epidermidis , hominis , lugdunensis , and pseudintermedius ) were downloaded from NCBI. The 6-TG operon and its homologs were identified using tBLASTn [50] using translation table 11 , with the S. chromogenes 6-TG operon used as the query sequence. Genomes that contained the operon are listed in Supplementary Data 1 . The 6-TG operon and its homologs were extracted, and their nucleotide sequences were aligned in Geneious Prime 2020.1.2 ( https://www.geneious.com ) using the Geneious aligner and the default settings. The alignment was used to create a phylogeny with RAxML using the rapid bootstrapping and search for best maximum likelihood tree algorithm with 1000 bootstrap iterations [51] . The RAxML tree was condensed with MEGA7 [52] using a bootstrap support cut-off of 50%. Three isolates possessed split 6-TG operons and were excluded from the phylogenetic analysis to minimize potential problems due to operon assembly. Cloning of the 6-TG biosynthetic cluster from S. chromogenes and S. capitis into S. aureus Genomic DNA was isolated from S. chromogenes and S. capitis by phenol–chloroform extraction. 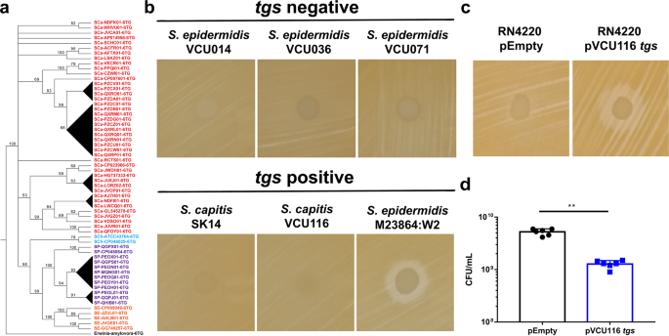Fig. 3: Thetgsoperon is present in other staphylococcal species and functional. aPhylogenetic analysis of the 6-TG operon using completed and draftStaphylococcusgenomes. Black triangles represent a clade that was collapsed because their internal bootstrap values were <50%. SCaS. capitis, SChS. chromogenes, SES. epidermidis, SPS. pseudintermedius.bSimultaneous antagonism assay oftgs-negative and -positive staphylococcal strains on TSA.cSimultaneous antagonism assay using RN4220 pEmpty and pVCU116tgson TSA.dS. aureuswas cultured in TSB containing supernatant from RN4220 pEmpty or pVCU116tgsand plated 24 h.p.i and CFU/mL were enumerated. Results are pooled from two independent experiments, each withn= 3 replicates per condition. Data are shown as mean ± SD (**p≤ 0.01. Two-sided unpairedt-test). Primers containing a KpnI or SacI restriction site were used to amplify the putative 6-TG biosynthetic cluster (TTTTTTGGTACCCCGAACTTTTATTCGAAAAT and TTTTTTGAGCTCCTAGTTTTTAATTGTAAAAC) from S. chromogenes ATCC43764 and (TTTTTTGGTACCTGTTTCTTTTACTTGTCTGC and TTTGAGCTCGGTTATTTTCAGTACACTCC) from S. capitis VCU116 (Supplementary Table 3 ). The amplified product was ligated into pALC2073 that was similarly digested and transformed into E. coli . Plasmids isolated from E. coli were introduced into S. aureus RN4220. Simultaneous antagonism and disc diffusion assays The OD 600 of bacteria was normalized to 1.0. Sterile cotton swabs were used to spread plate a suspension of the culture onto solid media. For simultaneous antagonism assays, 10 μL of overnight bacterial cultures were inoculated onto the bacterial lawn. 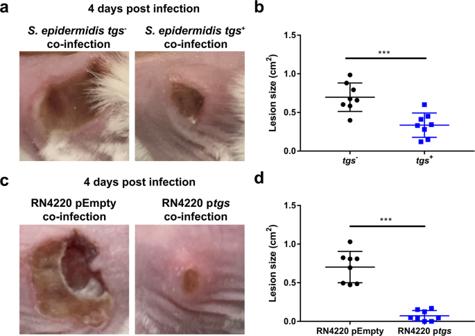Fig. 4:tgsexpressing staphylococci reduce skin damage caused byS. aureusduring co-infection. aRepresentative images showing necrotic skin lesions 4 days post infection withS. aureus+tgs-negativeS. epidermidisstr. VCU036 orS. aureus+tgs-positiveS. epidermidisstr. M23864:W2 in a 1:1 ratio.bQuantitation of necrotic skin lesion size 4 days post infection withS. aureus+tgs-negativeS. epidermidisstr. VCU036 orS. aureus+tgs-positiveS. epidermidisstr. M23864:W2 in a 1:1 ratio. Results are from one representative experiment enumerating 8 lesions per group (n= 4 animals per group). Data are shown as mean ± SD (***p≤ 0.001. Two-sided unpairedt-test).cRepresentative images showing necrotic skin lesions 4 days post infection withS. aureus+ RN4220 pEmpty orS. aureus+ RN4220 ptgsin a 1:1 ratio.dQuantitation of necrotic skin lesion size 4 days post infection withS. aureus+ RN4220 pEmpty orS. aureus+ RN4220 ptgsin a 1:1 ratio. Results are from one experiment enumerating 8 lesions per group (n= 4 animals per group). Data are shown as mean ± SD (***p≤ 0.001. Two-sided unpairedt-test). For modified simultaneous antagonism assays, a well in solid media was generated and 100 μL of a suspension was inoculated into the well. For disc diffusion assays, sterile paper discs were placed on top of the bacteria and 10 μL of 10-mg/mL 6-TG dissolved in 0.1-M NaOH was dropped onto the disc. For cinnamic acid, 10 μL of 10-mg/mL cinnamic acid was dissolved in 20% ethanol and dropped onto the disc. Plates were incubated at 37 °C overnight. Assessing the effect of the expression of the tgs operon on S. aureus growth kinetics Single colonies of RN4220 pEmpty, RN4220 p tgs and RN4220 pVCU116 tgs were inoculated into 5-mL TSB supplemented with chloramphenicol and grown overnight. Thirty milliliter of TSB supplemented with chloramphenicol were inoculated with bacteria from the overnight cultures such that the starting OD 600 was 0.01. The OD 600 of the cultures was measured every hour for the first 8 h. The OD 600 was then measured at the 12th and 24th hour post inoculation. Co-infections between S. aureus and tgs -positive and tgs -negative strains Eight-to-ten-week-old female Balb/c mice were shaved 1 day before the day of infection. Overnight cultures (grown in TSB) of S. aureus USA300, S. epidermidis str. VCU036, S. epidermidis str. M23864: W2, RN4220 pEmpty and RN4220 p tgs were subcultured to OD 600 of 0.05 in TSB and grown to OD 600 of 2.0–2.2. Bacterial cells were pelleted and washed in phosphate-buffered saline (PBS) twice. Bacterial cells were then normalized to the appropriate OD 600 and 25 μL of the S. aureus bacterial suspension (~5.0 × 10 7 CFUs) was mixed with 25 μL of the corresponding bacterial suspension (~5.0 × 10 7 CFUs for each strain) and subcutaneously injected into the animals. Infected mice were monitored daily for 4 days and sacrificed at 96 h post infection. Lesion sizes were analyzed in ImageJ. 6-TG prophylactic treatment of S. aureus subcutaneous skin infections Eight-to-ten-week-old female Balb/c mice were shaved and subcutaneously injected with 25 μL of 800 μg/mL 6-TG (equivalent to 20 μg 6-TG or 1 mg/kg) or a vehicle control 1 day before infection. This dosage was chosen based on the therapeutic concentration of 6-TG used in both mice and in humans for inflammatory bowel disease [53] , [54] . Overnight cultures (grown in TSB) of S. aureus USA300 were subcultured to OD 600 of 0.05 in TSB and grown to OD 600 of 2.0–2.2. Bacterial cells were pelleted and washed in PBS twice. Bacterial cells were then normalized to OD 600 3.7 and 25 μL of the bacterial suspension (~5.0 × 10 7 CFUs) were mixed with 25 μL of 800 μg/mL 6-TG and subcutaneously injected into the animals. Infected mice were monitored daily for 4 days and sacrificed at 96 h post infection. Lesions were excised in PBS with 0.1% (v/v) triton X-100, homogenized in a bullet blender tissue homogenizer (2 × 5 min at speed 6) and serially diluted before being plated onto TSA to enumerate CFUs. Lesion sizes were analyzed in ImageJ. Assessing the effect of 6-TG on S. aureus protein secretion by SDS-PAGE Single colonies of S. aureus grown on TSA were inoculated into TSB with 10-μg/mL 6-TG or a vehicle control and grown to an OD 600 of ~7.0–8.0. Proteins in the supernatant were harvested through trichloroacetic acid (TCA) precipitation. Briefly, supernatant derived from 6.0 OD 600 units of bacterial culture were mixed with an equal volume of ice-cold 20% (w/v) TCA for 3 h, washed twice with ice-cold 70% ethanol and air dried. The proteins were dissolved in 1x Laemmli SDS-PAGE reducing buffer and boiled for 10 min. Proteins were separated on a 12% SDS-PAGE gels and stained with InstantBlue TM Ultrafast Protein Stain overnight for visualization of protein bands. Assessing the effect of 6-TG on S. aureus alpha toxin by western blot Western blot analysis on alpha toxin was performed by transferring the SDS-PAGE gel to a nitrocellulose membrane. The membrane was then blocked with PBS supplemented with 0.1% (v/v) Tween 20 and 5% (w/v) milk. After blocking, the membrane was incubated with rabbit anti-Hla (1:500) polyclonal antibody (Sigma-Aldrich) for 2 h and washed with PBS-Tween 20 (3x). Donkey anti-rabbit IRDye 800 (1:20,000) (Rockland) was used as a secondary antibody for 45 min and the membrane was washed with PBS-Tween 20 (3x) prior to imaging. Membranes were scanned using an Odyssey Clx imaging system (Li-Cor Biosciences). Supernatants from both wild-type S. aureus and a Δ sbi Δ spa derivative were used, and the same results were obtained with either strain. Assessing the effect of 6-TG on S. aureus supernatant hemolysis Single colonies of S. aureus grown on TSA were inoculated into TSB. The overnight culture was subcultured into fresh TSB supplemented with a vehicle control or different concentrations of 6-TG. After 24 h of growth, the culture supernatants were centrifuged and filter-sterilized. Ten microliter of the cell-free supernatant was inoculated onto TSA supplemented with 5% (v/v) human red blood cells. Images were taken after 24 h and the area of the zone of hemolysis was measured using ImageJ. Assessing the effect of 6-TG on S. aureus growth kinetics Single colonies of S. aureus and S. aureus purK ::ΦΝΣ were inoculated into 5-mL TSB and grown overnight. Thirty milliliter of TSB with 10 μg/mL of 6-TG or a vehicle control were inoculated with bacteria from S. aureus or S. aureus purK ::ΦΝΣ overnight cultures such that the starting OD 600 was 0.01. The OD 600 of the cultures was measured every hour for 24 h. Preparation of cells for RNA extraction Single colonies of S. aureus and S. aureus purK ::ΦΝΣ were inoculated into 5-mL TSB and grown overnight. Five milliliter of TSB were inoculated with bacteria from S. aureus or S. aureus purK ::ΦΝΣ overnight cultures such that the starting OD 600 was 0.01. Cultures were grown until OD 600 = 1.0 (3–3.5 h) and 10-μg/mL 6-TG or a vehicle control was added to the culture. Cultures were grown for another hour. An equivalent of OD 600 = 6.0 of cells was collected and RNAprotect Bacteria Reagent (Qiagen) was mixed with the cells as per manufacturer’s instructions. Cell pellets were frozen overnight at −80 °C. RNA extraction and RNA-seq To extract RNA from frozen S. aureus and S. aureus purK ::ΦΝΣ, cell pellets were washed with TE buffer (pH 8.0) and re-suspended in a Tris-HCl mixture with 1-mg/mL lysostaphin (pH 7.5) to lyse for 1 h at 37 °C. RNA was extracted using an Aurum TM Total RNA Mini Kit (BioRAD #7326820) as per the manufacturer’s instructions. TURBO TM DNase (ThermoFisher Scientific) was used to cleave contaminating DNA, and RNA was further purified by phenol/chloroform extraction. Concentration and purity of RNA were determined using a Nanodrop. 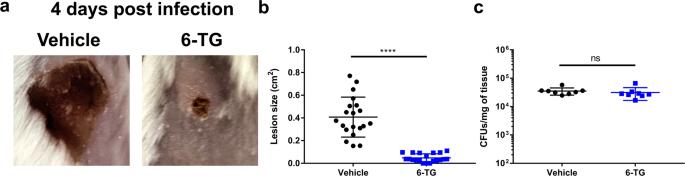Fig. 5: Prophylactic treatment with 6-TG reduces necrotic lesion size in subcutaneous infection. aRepresentative images showing necrotic skin lesions 4 days post infection withS. aureus± prophylactic 6-TG treatment.bQuantitation of necrotic skin lesion size 4 days post infection withS. aureus± prophylactic 6-TG (20 µg) treatment. Results are pooled from two independent experiments with 8–12 lesions per group (n= 4 and 6 animals, respectively). Data are shown as mean ± SD (****p≤ 0.0001. Two-sided unpairedt-test).cSkin tissue was excised from mice infected withS. aureus4 days post infection ± prophylactic 6-TG treatment (20 µg) and plated onto TSA to enumerate CFUs. Results are from one experiment with 8–12 lesions per group (n= 4 and 6 animals, respectively). Data are shown as mean ± SD (two-sided unpairedt-test). RNA samples were processed by the Microbial Genome Sequencing Center in Pittsburgh, PA. Ribosomal RNA was depleted (Qiagen FastSelect5S/16S/23S), and cDNA libraries were generated (Qiagen Total Stranded RNA). 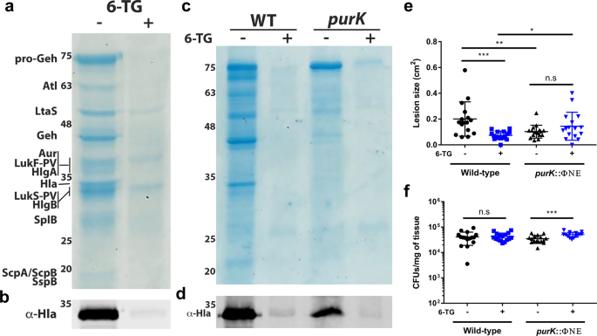Fig. 6: 6-TG reducesS. aureustoxin production in a purine-dependent and -independent manner. aS. aureuswas grown in the presence of 6-TG (10 µg/mL) or a vehicle control to an OD600of 7.0 and secreted proteins in the supernatant were TCA precipitated and separated by SDS-PAGE. This experiment was repeated three times with similar results.bProtein samples inawere immunoblotted and probed with anti-alpha toxin antibody in a Western blot. Protein identification was by MALDI TOF MS. Numbers indicate molecular mass markers. This experiment was repeated three times with similar results.cS. aureusandS. aureus purK::ΦΝΣ was grown in TSB with 6-TG (10 µg/mL) or a vehicle control to an OD600of 7.0 and secreted proteins in the supernatant were TCA precipitated and separated by SDS-PAGE. This experiment was repeated twice with similar results.dProtein samples incwere immunoblotted and probed with anti-alpha toxin antibody in a Western blot. This experiment was repeated twice with similar results.eQuantitation of necrotic skin lesion size 4 days post infection withS. aureusorS. aureus purK::ΦΝΣ ± prophylactic 6-TG (20 µg) treatment. Results are from one representative experiment with 16 lesions enumerated per group (n= 8 animals). Data are shown as mean ± SD (***p≤ 0.001, **p≤ 0.01, *p≤ 0.05. Two-sided unpairedt-test).fSkin tissue was excised from mice infected withS. aureusorS. aureus purK::ΦΝΣ 4 days post infection ± prophylactic 6-TG (20 µg) treatment and plated onto TSA to enumerate CFUs. Results are from one representative experiment with 16 lesions enumerated per group (n= 8 animals). Data are shown as mean ± SD (***p≤ 0.001. Two-sided unpairedt-test). Fora–d, numbers to the left of gels/blots are molecular mass markers (in kDa). 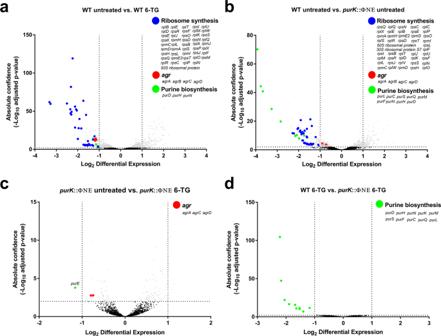Fig. 7: 6-TG abrogates toxin production by reducing transcription from the agr locus and from genes encoding for ribosomal proteins. aRNA-seq analysis of wild-typeS. aureuscultures treated with a vehicle control or 6-TG (10 µg/mL) in TSB. Data points above the dashed lines along thex-axis representp≤ 0.01. Data points outside of the dashed lines along they-axis represent fold changes of ≥2.0. Results are from four independent experiments.bRNA-seq analysis ofS. aureus purK::ΦΝΣ cultures treated with a vehicle control compared to wild-typeS. aureuscultures treated with a vehicle control in TSB. Results are from four independent experiments.cRNA-seq analysis ofS. aureus purK::ΦΝΣ cultures treated with a vehicle control or 6-TG (10 µg/mL) in TSB. Results are from four independent experiments.dRNA-seq analysis of wild-typeS. aureuscultures andS. aureus purK::ΦΝΣ cultures treated with 6-TG (10 µg/mL) in TSB. Results are from four independent experiments. Statistical significance was determined using a negative binomial distribution. Detailed RNA-seq data can be found in Supplementary Data2. cDNA libraries were sequenced using NextSeq 550 using a 75 × 8 × 8bp setup. Bioinformatic analyses of RNA-seq data Sequencing reads were mapped to the reference S. aureus USA300 FPR3757 genome in Geneious Prime 2020.1.2 ( https://www.geneious.com ). Expression analysis and comparisons were performed using DESeq2 [55] . Graphical and statistical analyses Statistical analyses were performed using GraphPad Prism software version 7. Statistical significance was calculated using ANOVA and Student’s t tests with SD as appropriate. Ethics approval All experiments involving animals were reviewed and approved by the Animal Use Subcommittee of the University of Western Ontario and were performed according to the Canadian Council on Animal Care guidelines. Reporting summary Further information on research design is available in the Nature Research Reporting Summary linked to this article.